What is and what is not electromagnetically induced transparency in whispering-gallery microcavities There has been an increasing interest in all-optical analogues of electromagnetically induced transparency and Autler–Townes splitting. Despite the differences in their underlying physics, both electromagnetically induced transparency and Autler–Townes splitting are quantified by a transparency window in the absorption or transmission spectrum, which often leads to a confusion about its origin. While the transparency window in electromagnetically induced transparency is a result of Fano interference among different transition pathways, in Autler–Townes splitting it is the result of strong field-driven interactions leading to the splitting of energy levels. Being able to tell objectively whether an observed transparency window is because of electromagnetically induced transparency or Autler–Townes splitting is crucial for applications and for clarifying the physics involved. Here we demonstrate the pathways leading to electromagnetically induced transparency, Fano resonances and Autler–Townes splitting in coupled whispering-gallery-mode resonators. Moreover, we report the application of the Akaike Information Criterion discerning between all-optical analogues of electromagnetically induced transparency and Autler–Townes splitting and clarifying the transition between them. Coherent interactions of light with multilevel atoms can dramatically modify their optical response via quantum interferences between various excitation pathways, or via strong-coupling-field-induced energy level splitting. The process known as electromagnetically induced transparency [1] , [2] , [3] , [4] (EIT) is the result of Fano interferences [5] , [6] that require coupling of a discrete transition to a continuum. EIT creates a narrow transparency window by eliminating a resonant absorption. EIT has a rich variety of applications such as ultraslow light propagation [7] , light storage [8] , [9] , dissipation-free light transmission and nonlinear optics with weak light. Autler–Townes splitting [10] (ATS) involves field-induced splitting of energy levels and is not associated with interference effects; yet it creates a transparency window because of the doublet structure in the absorption profile. It has been used for measuring transition dipole moments [11] and quantum control of spin–orbit interactions [12] . Coherent processes leading to EIT and ATS have been studied in: atomic gases [7] , [13] , atomic and molecular systems [14] , solid-state systems [15] , superconductors [16] , [17] , plasmonics [18] , metamaterials [19] , optomechanics [20] , [21] , electronics [22] , photonic crystals [23] and whispering-gallery-mode microresonators (WGMRs) [24] , [25] , [26] , [27] , [28] , [29] , [30] , [31] , [32] , [33] . Systems in which EIT and ATS have been studied are listed in Fig. 1 . Using the identifications listed in Fig. 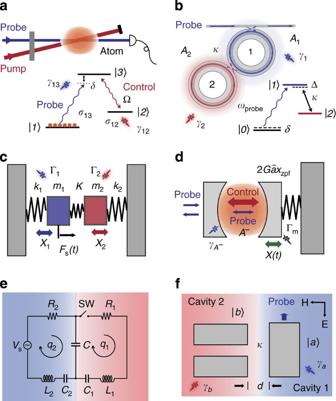Figure 1: Different platforms used for realizing electromagnetically induced transparency. (a) Atomic ensembles with Λ-type three-level atoms: ground state |1›; dark state |2›; excited state |3›; density matrix elementsσ12andσ13; pump field Rabi frequency Ω; dephasing ratesγ12andγ13; detuningδ(ref.17). (b) Coupled system of microresonators: intracavity field amplitudesA1andA2; cavity coupling strengthκ; decay ratesγ1andγ2of the optical modesA1andA2; resonance detuning Δ; detuning of the probe fieldδ(ref.24). (c) Mechanical systems: spring constantsK,k1,k2; massesm1andm2; displacementsX1andX2of mass 1 and mass 2, respectively; mechanical dampings Γ1and Γ2; driving forceFs(t) (ref.22). (d) Optomechanical systems: intracavity field amplitudeA−; mechanical displacementX; optomechanical coupling strength 2Gāxzpf; decayofA−; mechanical damping Γm(ref.20). (e) Electronic circuits: inductorsL1andL2; capacitorsC,C1andC2; resistorsR1andR2; voltage sourceVs; chargesq1andq2in the resonance circuits; switch SW (ref.22). (f) Plasmonics: the radiative plasmonic state |a›; the dark plasmonic state |b›; plasmonic coupling strengthκ; damping ratesγaandγb(ref.18). Correspondences and analogies among these system-specific parameters are shown inTable 1. 1 and Table 1 , it can be easily shown that equations and relations describing the EIT and ATS in one of these systems are equivalent to those in the others. The existence of EIT and ATS in plasmonics, metamaterials, photonic crystals and WGMRs is critical for on-chip control of light at room temperature. EIT and ATS in these systems do not suffer from experimental complexities that are common in solid state and atomic media (for example, a low-temperature environment, the need for stable lasers matching the atomic transitions or propagation-scaling limitations because of control-field absorption). Figure 1: Different platforms used for realizing electromagnetically induced transparency. ( a ) Atomic ensembles with Λ-type three-level atoms: ground state |1›; dark state |2›; excited state |3›; density matrix elements σ 12 and σ 13 ; pump field Rabi frequency Ω; dephasing rates γ 12 and γ 13 ; detuning δ (ref. 17 ). ( b ) Coupled system of microresonators: intracavity field amplitudes A 1 and A 2 ; cavity coupling strength κ ; decay rates γ 1 and γ 2 of the optical modes A 1 and A 2 ; resonance detuning Δ; detuning of the probe field δ (ref. 24 ). ( c ) Mechanical systems: spring constants K , k 1 , k 2 ; masses m 1 and m 2 ; displacements X 1 and X 2 of mass 1 and mass 2, respectively; mechanical dampings Γ 1 and Γ 2 ; driving force F s ( t ) (ref. 22 ). ( d ) Optomechanical systems: intracavity field amplitude A − ; mechanical displacement X ; optomechanical coupling strength 2 Gāx zpf ; decay of A − ; mechanical damping Γ m (ref. 20 ). ( e ) Electronic circuits: inductors L 1 and L 2 ; capacitors C , C 1 and C 2 ; resistors R 1 and R 2 ; voltage source V s ; charges q 1 and q 2 in the resonance circuits; switch SW (ref. 22 ). ( f ) Plasmonics: the radiative plasmonic state | a ›; the dark plasmonic state | b ›; plasmonic coupling strength κ ; damping rates γ a and γ b (ref. 18 ). Correspondences and analogies among these system-specific parameters are shown in Table 1 . Full size image Table 1 Correspondences among parameters of various systems ( Fig. 1 ) in which EIT and ATS have been experimentally observed. Full size table WGMRs have been a fruitful platform to study various aspects of classical and all-optical analogues of EIT and ATS. Fano resonances and EIT have been observed in a silica microsphere [28] , a polydimethyl-siloxane-coated silica microtoroid with two WGMs [29] , two directly coupled silica microspheres [25] , [30] , two indirectly coupled silicon microrings [26] , and indirectly coupled microdisk and microtoroid [31] . In these EIT implementations, two frequency-degenerate WGMs of high- and low-quality factors (Q) are coupled, and destructive interference of the optical pathways cancels the absorption leading to a narrow transmission peak. If a frequency detuning is introduced, the transmission spectra show sharp asymmetric Fano resonances. ATS has been observed in directly coupled silica microspheres [25] , directly coupled silica microtoroids [34] , hybrid systems formed by directly coupling polydimethyl-siloxane-coated silica microtoroids with silica microtoroids or microspheres [35] and directly coupled polyethylene and quartz disks in the THz domain [36] . In these systems, ATS originates from the lifting of the frequency degeneracy of the eigenmodes, hence their splitting into two resonances because of strong inter-resonator coupling. The spectral region between the split modes corresponds to a transparency window. A scatterer-induced coupling between the frequency-degenerate clockwise and counter-clockwise travelling modes of a WGMR can also lead to mode-splitting [37] , [38] , [39] . This has been used to detect and measure nanoscale objects with single particle resolution [37] and to directly measure the Purcell factor [40] . The effects of ATS in the absorption profile resemble that of EIT, in that both of the processes display a transparency window, that is, a reduction in the absorption profile. This similarity has led to much confusion [16] , [41] , [42] and many discussions [17] , [43] , [44] , [45] , [46] on how to discriminate between EIT and ATS just by looking at the experimentally obtained absorption/transmission spectra, without prior knowledge on the system. The sharpness of the dip in the absorption and the imaginary part of the susceptibility (or the peak in the transmission) has been used as an intuitive and informal criterion to judge whether EIT takes place or not. However, such a test is very subjective. For example, a peak in the transmission spectrum is in general much sharper than the dip in the absorption spectrum of the same system. Therefore, one has to first decide whether to focus on the sharpness of the transmission or the sharpness of susceptibility/absorption. Moreover, system-specific parameters affect the output spectra. Namely, relaxation rates, coupling strengths and cleanliness of the samples differ among different systems and determine the sharpness of the spectrum. For example, these parameters in superconducting systems are at least one to two orders-of-magnitude less than their atomic counterparts; hence, the dip in the susceptibility of superconducting systems is lesser sharp than that of alkaline atoms [47] . Therefore, objective and system-independent methods and tests are needed to make claims of EIT. Since identifying whether an experiment involves EIT or ATS is important for applications, objective methods to discriminate between them have been sought. Many studies have been carried out to identify the conditions to observe EIT or ATS [43] , [44] , [45] , [46] , [47] . Recently Anisimov et al. [17] have proposed to use the Akaike Information Criterion (AIC) [48] as an objective test to discern EIT from ATS in experimentally obtained absorption or transmission spectra, and to identify the spectra from which one cannot derive a conclusive result on whether EIT or ATS has played a role. They have successfully applied this test to an experiment with a one-dimensional (1D) superconducting transmission line coupled to a flux qubit, concluding that the reported data [16] do not support the claim of EIT. In a recent study, Giner et al. [49] demonstrated the suitability of the AIC criterion to evaluate EIT and ATS in experiments with cold caesium atoms. Oishi et al. [50] suggested that the transient response of a system can be used to discern EIT from ATS. The transient response exhibits a sharp spike when the system is prepared for EIT; however, when it is prepared for ATS, an oscillatory signal attributed to coherent energy exchange between the resonators is observed. Note that AIC discriminates EIT from ATS in the frequency domain, whereas the transient response method discriminates them in the time domain. Up to this date, there was no study to discern EIT from ATS in coupled optical WGMRs. Here we systematically investigate Fano resonances, EIT and ATS in coupled microtoroids, identify the transition from EIT to ATS (and vice versa ) and use AIC to discern EIT from ATS from experimentally obtained transmission spectra. Our results show the suitability of the AIC for discriminating EIT from ATS in systems of coupled WGMRs. Experimental set-up Our system consists of two directly coupled silica microtoroidal WGM resonators μR1 and μR2, with μR1 coupled to a fibre taper ( Fig. 2 ). We fabricated the silica microtoroids at the edges of two separate silicon wafers, such that when the wafers were brought closer to each other, the microtoroids began exchanging energy. The wafers were placed on separate nanopositioning systems so that the distance between the microtoroids was finely tuned to control the coupling strength κ between them. The coupling strength κ decreases exponentially with increasing distance. The probe light in the 1,550-nm band from a narrow linewidth tunable laser was coupled into a WGM of μR1 via the fibre taper. The same fibre taper was also used to couple out the light from the WGM. The output light was then sent to a photodetector connected to an oscilloscope, to obtain the transmission spectra as the wavelength of the input light was linearly scanned. Fibre-based polarization controllers were used to set the polarization of the input light for maximal coupling into WGMs. A thermoelectric cooler was placed under one of the wafers so that resonance frequency of the WGM of interest in a microtoroid could be tuned via the thermo-optic effect, to control the frequency detuning of the chosen WGMs in the two microtoroids. A tuning range of 8 GHz was achieved. The microtoroids supported many WGMs in the same band but with different quality factors Q, which is the signature of the amount of loss or dissipation (the lower the loss, the higher the Q and the narrower the linewidth of the resonance mode). This allowed us to investigate the effects of Q of the selected modes on the Fano, EIT and ATS processes by choosing WGM pairs with different Q-contrasts. In addition to the ability of choosing different WGM pairs, our set-up allowed us to investigate Fano, EIT and ATS processes and the transitions among them by steering the system independently via the coupling strength or the frequency detuning between the selected WGMs. In our experiment, we selected three different sets of WGM pairs with the intrinsic quality factors ( Q μR1 and Q μR2 ) of (1.91 × 10 5 , 7.26 × 10 7 ), (1.63 × 10 6 , 1.54 × 10 6 ) and (1.78 × 10 6 , 4.67 × 10 6 ). Note that the intrinsic Q includes all the losses (for example, material, radiation and scattering) except the coupling losses. Since the probe light is input at the μR1 side with a fibre taper, the Q of the μR1 is smaller than the above intrinsic Q-values because of the additional coupling losses (that is, μR1 has more loss than μR2). 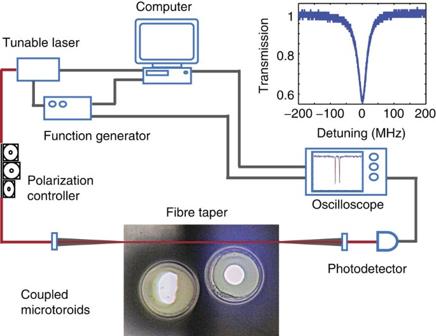Figure 2: Experimental configuration for the coupled WGM microcavity system. Set-up with a microscope image of the coupled microtoroid system. The system consists of two directly coupled WGM resonators (μR1 and μR2), and a fibre taper waveguide coupled to μR1. The probe laser is in the 1,550-nm band. Inset: typical transmission spectra showing the resonant mode in μR1. Figure 2: Experimental configuration for the coupled WGM microcavity system. Set-up with a microscope image of the coupled microtoroid system. The system consists of two directly coupled WGM resonators (μR1 and μR2), and a fibre taper waveguide coupled to μR1. The probe laser is in the 1,550-nm band. Inset: typical transmission spectra showing the resonant mode in μR1. Full size image Analogy between coupled resonators and three-level atoms Here we will elucidate the analogy between atomic and photonic coherence effects leading to EIT and ATS. Using coupled-mode theory, we find the equations of motion for the complex intracavity field amplitudes A 1 and A 2 in the steady state as where and γ 2 denote the total losses in μR1 and μR2, respectively, is the intrinsic loss of μR1 and γ c is the coupling loss between the fibre taper and μR1, δ 1 = ω − ω 1 and δ 2 = ω − ω 2 denote the detuning between the frequency ω of the probe light field A p and the resonance frequencies ω 1 and ω 2 of the WGMs, and κ is the coupling strength between the WGMs. In the EIT and ATS experiments, we set ω 1 = ω 2 = ω 0 via the thermo-optic effect by thermally tuning the frequency of one of the WGMs to be equal to the frequency of the other. Consequently, for the degenerate frequencies ω 1 and ω 2 we have Δ= ω 2 − ω 1 =0, and in the rotated frame ( ω 0 →0) we have δ 1 = δ 2 = ω . In addition, note that in the system depicted in Figs 1b and 2 the input and output ports are at the side of μR1; hence, the output field is given as where the intracavity field A 1 can be written as with where we used α k = iω k + γ k /2, with k =1, 2. This solution χ has a form similar to the response of an EIT medium (three-level atom) to a probe field. Then, we can write the normalized transmission T =| A out / A p | 2 as where χ i is the imaginary part of χ. Since and we can rewrite the transmission as Thus, it is sufficient to analyse the behaviour of χ i to understand the conditions leading to EIT or ATS ( Supplementary Note 1 ). This is similar to considering the imaginary part of the susceptibility that determines the absorption of a probe in an atomic system. This analogy between the atomic media and the coupled WGMRs can be extended to other systems by using the analogy map given in Fig. 1 and Table 1 . The eigenfrequencies of this coupled system can be found from the denominator of equation (3) and are given as ω ± =(− iα 1 − iα 2 ± β )/2, with β 2 =4 κ 2 −( α 1 − α 2 ) 2 . This reveals a transition at the threshold coupling strength 2| κ T |= α 1 − α 2 =( γ 1 − γ 2 )/2, where we have used the fact that in our system γ 1 > γ 2 , as stated in the previous section. We define the regimes where κ < κ T and κ > κ T as the weak- and strong-driving regimes, respectively, and κ = κ T as the transition point. Using the eigenfrequencies, we can rewrite the expression in equation (3) as where χ ± = ∓ ( ω ± + iα 2 )/ β =−1/2± iξ / β satisfying χ + + χ − =−1 and ξ =( γ 1 − γ 2 )/4. In the weak-driving regime quantified by κ < κ T , β is imaginary, that is β = iβ i and Re( β )= β r =0. This leads to real χ ± (that is, Im( χ ± )= χ ±i =0) with Re( χ ± )= χ ±r =−1/2± ξ /| β |, and imaginary eigenfrequencies with Re( ω ± )= ω ±r =0 and Im( ω ± )= ω ±i =− ζ ±| β |/2, where ζ =( γ 1 + γ 2 )/4. Thus, the supermodes have the same resonance frequencies and are located at the centre of the frequency axis but have different linewidths quantified by their imaginary parts. The imaginary parts of χ are then given by which consists of two Lorentzians centred at ω =0 with different signs (that is, the first term in the equation is negative, whereas the second term is positive). The transmission in this regime becomes where all the parameters whose values cannot be determined precisely are incorporated into the coefficients C k and Γ k that can be used as free parameters to perform curve-fitting to experimentally obtained transmission spectra. Clearly, the opposite signs of the Lorentzians lead to a destructive interference that results in a transmission profile exhibiting a transparency window similar to that of EIT. In the strong-driving regime, where κ >> κ T is satisfied, β =2 κ is real (that is, β i =0 and β r =2 κ ) implying ω ± =− iζ ± κ , that is the resonances are located at frequencies ± κ with a spectral distance of 2 κ between them. The resonance linewidths are quantified by Im( ω ±)=− ζ . Approximating χ ± as χ ± =−1/2 we find the imaginary part of χ as which implies that χ i is the sum of two same-sign Lorentzians centred at ± κ . The transmission in this regime is then given by where C , Γ and δ are the free parameters that can be used in curve-fitting to experimentally obtained transmission spectra. Clearly, the transmission in this strong-driving regime presents a symmetric doublet spectra and the observed transparency is because of the contribution of two Lorentzians. In the intermediate-driving regime [51] quantified by κ > κ T , β = β r is real (that is, β i =0). This leads to complex eigenfrequencies ω ± =(− iγ 1 − iγ 2 ±2 β r )/4 and complex χ ± =−1/2± i ( γ 1 − γ 2 )/4 β r . Thus, the supermodes have different resonance frequencies located at ± β r /2 but have the same linewidths quantified by their imaginary parts Im( ω ± )= ω ±i =(− γ 1 − γ 2 )/4. Consequently, we have and where ε = β r /2. The expression in the second bracket of equation (12) is the sum of two Lorentzians, similar to the expression obtained for the strong-driving regime in equation (10), implying the contribution of ATS. The expression in the first bracket corresponds to the interference term and can be controlled by choosing the loss of the coupled modes. For example, choosing two modes satisfying γ 1 = γ 2 will lead to C 1 =0, and hence the expression T EIT/ATS will become the same as T ATS . This implies that to observe ATS, the linewidths (that is, Q) of the coupled WGMs should be very close to each other as will be demonstrated in the experiments discussed below. The theoretical shapes and more detailed discussions of these operating regimes are given in Supplementary Note 1 and Supplementary Figs 1–3 . Fano resonances and EIT in experiments with coupled WGMRs EIT is a result of strong Fano interferences and takes place when a high-Q WGM of one microresonator is directly coupled to a low-Q WGM of a second microresonator with zero-detuning in their resonance frequencies. In order to demonstrate this, we chose a low-Q mode in μR1 ( Q μR1 =1.91 × 10 5 ) and a high-Q mode in μR2 ( Q μR2 =7.26 × 10 7 ). We then set the distance between the resonators such that the coupling strength was smaller than the loss contrast of the resonators. At this point, we continuously tuned the frequency of the high-Q mode in μR2 such that it approached to the frequency of the low-Q mode in μR1. As the frequency-detuning between the modes gradually decreased, the modes became spectrally overlapped. Consequently, we first observed an asymmetric Fano lineshape with the peak located closer to the lower-detuning side ( Fig. 3a , upper panels), and then a transparency window appeared at zero-detuning ω 2 − ω 1 =0 ( Fig. 3a , middle panel). The linewidth of the transparency window was 5 MHz. The asymmetry of Fano resonances decreased as we approached to zero-detuning. As the frequency of the high-Q mode was further increased, detuning started to increase again leading to the emergence of Fano lineshapes whose peaks were also located closer to zero-detuning ( Fig. 3a , lower panels). Finally, when the frequency was increased such that there was no overlap between the modes, Fano lineshapes were lost and we observed two independent Lorentzian lineshapes corresponding to the two modes in μR1 and μR2. 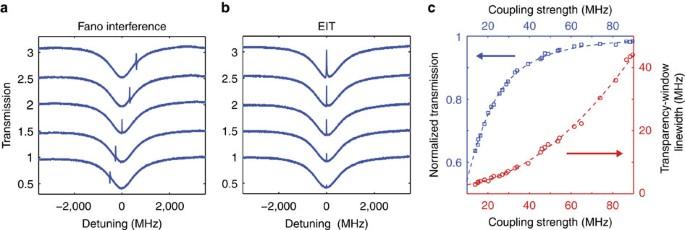Figure 3: Fano interference and EIT in coupled WGM microcavities. (a) Spectral tuning of the system from asymmetric Fano resonance to EIT. When the resonance modes of the microresonators have non-zero frequency-detuning, the transmission exhibits asymmetric Fano resonances. At zero detuning, a transparency window appears. (b) Effect of coupling strength on the EIT spectra (that is, zero detuning between resonance modes of the resonators). The coupling strength (increasing from the bottom to the top curve) depends on the distance between the resonators. (c) Effect of the coupling strength on the linewidth (red circles) and the peak transmission (blue squares) of the transparency window. The curves are the best fit to the experimental data. Figure 3: Fano interference and EIT in coupled WGM microcavities. ( a ) Spectral tuning of the system from asymmetric Fano resonance to EIT. When the resonance modes of the microresonators have non-zero frequency-detuning, the transmission exhibits asymmetric Fano resonances. At zero detuning, a transparency window appears. ( b ) Effect of coupling strength on the EIT spectra (that is, zero detuning between resonance modes of the resonators). The coupling strength (increasing from the bottom to the top curve) depends on the distance between the resonators. ( c ) Effect of the coupling strength on the linewidth (red circles) and the peak transmission (blue squares) of the transparency window. The curves are the best fit to the experimental data. Full size image Next, we studied the effect of coupling on the transparency window by first setting the frequency detuning of the low- and high-Q modes to zero, and then tuning the distance between the microtoroids ( Fig. 3b ). Note that the coupling strength here corresponds to the strength of the control field in atomic systems. We observed that as the coupling strength was increased (that is, the distance between the microtoroids decreased) the transmission at the transparency window increased from 0.63 to 0.98 ( Fig. 3c ). During this process, the linewidth of the transparency window increased from 3 to 43 MHz ( Fig. 3c ). Experimental demonstration of ATS in coupled WGMRs Contrary to EIT, ATS is not a result of Fano interferences but requires a strong-coupling between two WGMs of similar Q. In order to demonstrate this, we chose the mode with Q μR1 =1.63 × 10 6 in μR1 and the mode Q μR2 =1.54 × 10 6 in μR2. We first tuned the resonance frequencies of the modes to have ω 1 = ω 2 (that is, zero-detuning) when the microtoroids were sufficiently away from each other so that they could not exchange energies (that is, no coupling). At this stage, the transmission showed single resonance with Lorentzian lineshape ( Fig. 4a , lowest panel). As we started to bring the resonators closer to each other (that is, increased coupling strength), the single resonance split into two resonances whose spectral distance (that is, mode splitting) increased with increasing coupling strength. For large coupling strengths, the transmission spectra were well-fitted by two Lorentzian resonances. 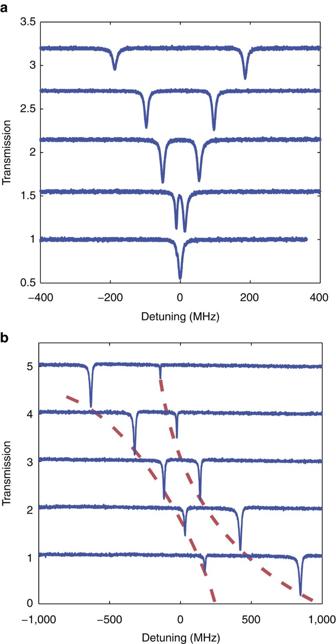Figure 4: ATS and avoided crossing in coupled WGM microcavities. (a) Effect of the coupling strength on the ATS spectra. During the process, the resonance modes had zero frequency detuning, and as the coupling strength was increased (from the bottom to the top curve) the splitting increased. (b) Effect of the frequency detuning of the coupled resonant modes on the ATS spectra. When the two resonant modes had non-zero detuning, the transmission exhibited asymmetric ATS (unequal transmission dips). As the frequency of one of the resonant modes was increased (frequency detuning approaches zero), the split modes started to approach each other and the transmission exhibited more symmetric ATS spectrum. With further increase in the frequency, the split modes exhibited avoided crossing. The smallest splitting was ~300 MHz, at which the frequency detuning between the resonant modes was zero. Further increase in the resonance frequency then led back to an asymmetric ATS. Figure 4: ATS and avoided crossing in coupled WGM microcavities. ( a ) Effect of the coupling strength on the ATS spectra. During the process, the resonance modes had zero frequency detuning, and as the coupling strength was increased (from the bottom to the top curve) the splitting increased. ( b ) Effect of the frequency detuning of the coupled resonant modes on the ATS spectra. When the two resonant modes had non-zero detuning, the transmission exhibited asymmetric ATS (unequal transmission dips). As the frequency of one of the resonant modes was increased (frequency detuning approaches zero), the split modes started to approach each other and the transmission exhibited more symmetric ATS spectrum. With further increase in the frequency, the split modes exhibited avoided crossing. The smallest splitting was ~300 MHz, at which the frequency detuning between the resonant modes was zero. Further increase in the resonance frequency then led back to an asymmetric ATS. Full size image Next, we chose two detuned resonance lines and set the coupling to strong-coupling regime (that is, resonators are very close to each other). We observed that the split modes in the transmission were not symmetric ( Fig. 4b , upper panel), and they had different transmission dips. This can be attributed to the unequal distribution of the supermodes in the two resonators. As we tuned the spectral distance between the WGMs by increasing the frequency of the mode in μR2, the split modes started to approach each other (that is, decreasing mode-splitting) and the difference between their transmission dips decreased. At zero-detuning the resonances became symmetric, that is they are Lorentzian with the same linewidths and transmission dips ( Fig. 4b , middle panel). Here the supermodes are equally distributed between the resonators. When the frequency of the mode in μR2 was further increased beyond the zero-detuning point, the modes repelled each other leading to an avoided crossing during which they interchanged their linewidths and transmission dips ( Fig. 4b , lower panels). Discerning EIT from ATS using AIC As we have discussed in the previous sections, in the theoretical model and the experimental observations, EIT and ATS both display a transparency window in the transmission spectrum of coupled microresonators (that is, similar to a three-level quantum system). However, EIT is because of Fano interference and hence requires coupling between a high-Q mode (that is, discrete system) and a low-Q mode (that is, continuum) in the weak-driving regime, while ATS is because of strong-coupling induced splitting of resonance modes and requires the interaction between modes with similar Q in the strong-driving regime. Thus, depending on the relative Q’s of the interacting modes and their coupling strength, the system of coupled microresonators can operate in either the EIT or the ATS regimes. Discerning whether a transparency window in the transmission spectrum of the system of coupled resonators is the signature of EIT or ATS without a priori information on the Qs and coupling strength between the modes is crucial. Here we performed experiments under various conditions of our coupled-resonator system, obtained transmission spectra and used the AIC proposed to discriminate between EIT and ATS in atomic systems to discern EIT or ATS. The AIC provides a method to select the best model from a set of models based on the Kullback–Leibler (K–L) distance between the model and the truth. The K–L distance quantifies the amount of information lost when approximating the truth. Thus, a good model is the one that minimizes the information loss and hence the K–L distance. Then AIC quantifies the amount of information lost when the model λ i with k i unknown parameters out of N models is used to fit the data x = x 1 , x 2 , ..., x n obtained in the measurements, and is given as I i =−2log L i +2 k i , where L i is the maximum likelihood for the candidate model λ i and 2 k i accounts for the penalty for the number of parameters used in the fitting. Then, the relative likelihood of the model λ i is given by the Akaike weight . In the case of least-squares and the presence of technical noise in the experiments, a fitness test using per-point (mean) AIC weight , where Ī i = I i / n , can be applied. In our study involving only two models ( N =2), we can rewrite w i and as with w EIT + w ATS =1 and . In our experiments, we acquired 10,000 data points ( n =10,000) to form a transmission spectrum at each setting of coupling strength and frequency-detuning, and we repeated the measurements to obtain 10 transmission spectra at each setting, to take into account the fluctuations and uncertainty in the measurements. We used T EIT and T ATS given in equation (8) and equation (10), respectively, to fit the transmission spectra obtained in the experiments. Then we used the AIC tests proposed by Anisimov et al . [17] by calculating ( w EIT , w ATS ) and to determine which of the models (EIT or ATS) is the most likely for the experimental observation. In Fig. 5 , we present typical curves of ( w EIT , w ATS ) and obtained at three different experimental settings, corresponding to three different regimes of operation, as the coupling strength was increased: EIT-dominated ( Fig. 5a ), ATS-dominated ( Fig. 5b ) and EIT-to-ATS transition regime ( Fig. 5c ). The models assigned using AIC to the experimental data agree very well with the requirements to observe EIT or ATS. 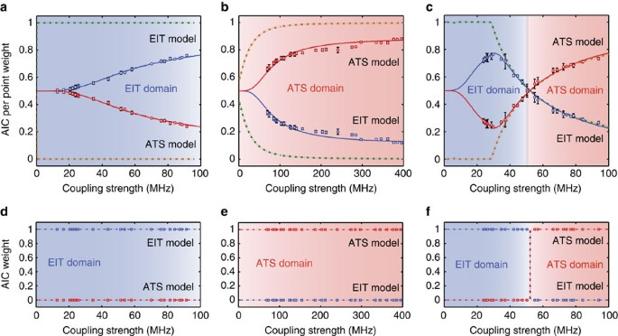Figure 5: AIC to discriminate EIT from ATS in optical microcavities. (a) The AIC per-point weight for the pair of modes chosen in the first and second microresonators with Q~(1.91 × 105, 7.26 × 107). As the coupling strength was increased, the EIT model dominated. (b) The AIC per-point weight for pair of modes with Q~(1.63 × 106, 1.54 × 106). As the coupling strength was increased above 60 MHz, the ATS model dominated. (c) The AIC per-point weight for the pair of modes with Q~(1.78 × 106, 4.67 × 106). A transition from EIT-dominated to ATS-dominated regime is clearly seen. (d–f) The AIC weights for the mode pairs studied in (a–c). Data for EIT and ATS are given in blue and red marks/curves, respectively, and the green and orange marks/curves represent the theoretical AIC per-point weights (that is, these do not take into account the experimental noise). Each data point is the average of 10 measurements, and the error bars represent the s.d.’s. Figure 5: AIC to discriminate EIT from ATS in optical microcavities. ( a ) The AIC per-point weight for the pair of modes chosen in the first and second microresonators with Q~(1.91 × 10 5 , 7.26 × 10 7 ). As the coupling strength was increased, the EIT model dominated. ( b ) The AIC per-point weight for pair of modes with Q~(1.63 × 10 6 , 1.54 × 10 6 ). As the coupling strength was increased above 60 MHz, the ATS model dominated. ( c ) The AIC per-point weight for the pair of modes with Q~(1.78 × 10 6 , 4.67 × 10 6 ). A transition from EIT-dominated to ATS-dominated regime is clearly seen. ( d – f ) The AIC weights for the mode pairs studied in ( a – c ). Data for EIT and ATS are given in blue and red marks/curves, respectively, and the green and orange marks/curves represent the theoretical AIC per-point weights (that is, these do not take into account the experimental noise). Each data point is the average of 10 measurements, and the error bars represent the s.d.’s. Full size image In the first case ( Fig. 5a ), the WGMs in the resonators were chosen such that their decay rates, quantified by Q μR1 (that is, γ 1 ) and Q μR2 (that is, γ 2 ), significantly differed from each other (that is, Q μR2 / Q μR1 ~400). We calculated κ T =| γ 1 − γ 2 |/4=312.8 MHz, which was larger than the coupling strengths used in the experiments ( κ <100 MHz). Starting from (that is, both the EIT and the ATS models are equally likely) for very weak coupling strength (0≤ κ ≤15 MHz ≪ κ T ), the likelihood of EIT model increased as the coupling strength was increased up to 100 MHz. Thus, we conclude that in this setting, which corresponded to weak-driving regime ( κ < κ T ), data obtained in the experiments favour the EIT model, as revealed by . In the second case ( Fig. 5b ), the decay rates of the coupled WGMs were very similar to each other (that is, Q μR2 / Q μR1 ~0.95), and we estimated the critical coupling strength as κ T =16.2 MHz, which was smaller than the coupling strengths considered κ >60 MHz. Therefore, as demonstrated in the model, this falls in the strong-driving regime ( κ >> κ T ), where ATS is expected. Indeed, in this experimental setting, starting from , the likelihood of the ATS model increased as the coupling strength was increased up to 400 MHz. Thus, the data obtained in the experiments favours the ATS model as revealed by . The third case ( Fig. 5c ) revealed an interesting phenomenon: transition from an EIT-dominated regime to an ATS-dominated regime through an inconclusive regime, where both EIT and ATS are equally likely. The decay rates of the chosen WGMs were similar (that is, Q μR2 / Q μR1 ~2.6); larger than that of the setting of Fig. 5b but much smaller than that of the setting in Fig. 5a . We estimated the critical coupling strength as κ T =29.5 MHz. In this case, the EIT model first dominated when the coupling strength was small. Then the likelihood of the EIT model decreased and that of the ATS model increased as the coupling strength was increased up to 50 MHz, where we observed . Further increase in the coupling strength beyond this point revealed a transition to an ATS-dominated regime . This results agree well with the predictions of the model: in the EIT-dominated regime we had κ < κ T , in the transition regime we had κ ~ κ T and finally in the ATS-dominated regime we had κ >> κ T . In Fig. 5d–f , we also present ( w EIT , w ATS ) as a function of the coupling strength. As expected, these weights exhibit a binary behaviour with an abrupt change from the EIT-dominated regime to the ATS-dominated regime. Since we collected 10 sets of data at each specific condition, we could assign s.d.’s to the AIC weights as seen in Fig. 5 . The technical noise in the experimental data points plays an accumulated role in the model fitting, which blurs the distinction between the models. This is clearly seen in the comparison of the AIC weights obtained from the experimental data with the theoretical weights. When the coupling strength was very small, in particular for the EIT regime, the noise had a larger blurring effect. This is attributed to the fact that in the very weak coupling regime, the EIT transparency window is so small that it is buried in the noise; thus, the contribution of the transparency band to the whole fitting decreases. The factors that affect the fitting and hence the model-assignment according to AIC weights are thermal noise, the probe laser frequency and amplitude fluctuations, the limited number of data points acquired for each spectrum, the resolution of the measurement equipments and the efficiency of the detector. We estimated that the s.d. of the total noise in our experiments is 1–2.5% of the measured signal. Finally in Fig. 6 we show examples of typical transmission spectra obtained in our experiments in the EIT-dominated ( Figs 5a and 6a ), the ATS-dominated ( Figs 5b and 6b ) and the EIT-to-ATS transition regimes ( Figs 5c and 6c ), together with the best-fitting curves using the expressions T EIT and T ATS derived from the theoretical model. It is clear that for the spectrum for which the AIC assigned the EIT model, the function T EIT provided a better fit than T ATS . In particular, the T ATS fitting performed poorly around the narrow transparency window ( Fig. 6a inset). In the spectrum for which the ATS model was assigned according to AIC weights, T ATS performed extremely well, whereas the T EIT fitting was very poor ( Fig. 6b ). The experimental conditions for the data shown in Fig. 5c revealed a transition from EIT to ATS. We chose a spectrum obtained in the vicinity of the transition point and performed curve-fitting using T EIT and T ATS . It is clearly seen in Fig. 6c that T EIT and T ATS functions perform equally well and one cannot conclusively assign a model to it: we cannot conclusively show EIT (or ATS) nor rule EIT (or ATS) out. These curve-fitting tests ( Fig. 6 ) agree well with the predictions of the AIC weights ( Fig. 5 ). 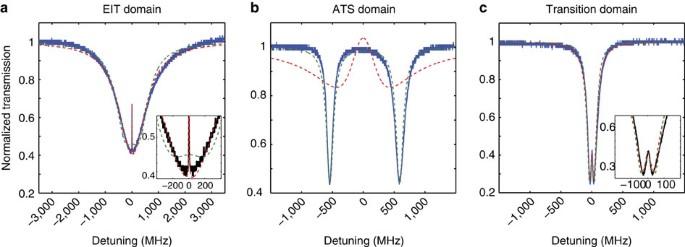Figure 6: Experimentally observed transmission spectra with EIT and ATS model fittings. The transmission spectra shown here are chosen to represent the three regimes (EIT-dominated, ATS-dominated and EIT-to-ATS transition regimes) observed inFig. 5according to AIC weights and per-point weights. Data obtained in the experiments are given in blue curves (black in the insets), and the best fits using theTEITmodel and theTATSmodel are given by the red and green curves, respectively. (a) The mode pair with Q~(1.91 × 105, 7.26 × 107) shows a clear transparency window, and the EIT model provides the best fit. This agrees with the result inFig. 5a,d. (b) The mode pair with Q~(1.63 × 106, 1.54 × 106) exhibits a broader transparency window with the best fit provided by the ATS model. This agrees with the result inFig. 5b,e. (c) At the transition region, both the EIT and the ATS models fit equally well to the transmission spectrum obtained for the mode pair with Q~(1.78 × 106, 4.67 × 106). This agrees well with the results ofFig. 5c,f. Insets are enlarged versions of the spectra around the central frequency (zero detuning). Figure 6: Experimentally observed transmission spectra with EIT and ATS model fittings. The transmission spectra shown here are chosen to represent the three regimes (EIT-dominated, ATS-dominated and EIT-to-ATS transition regimes) observed in Fig. 5 according to AIC weights and per-point weights. Data obtained in the experiments are given in blue curves (black in the insets), and the best fits using the T EIT model and the T ATS model are given by the red and green curves, respectively. ( a ) The mode pair with Q~(1.91 × 10 5 , 7.26 × 10 7 ) shows a clear transparency window, and the EIT model provides the best fit. This agrees with the result in Fig. 5a,d . ( b ) The mode pair with Q~(1.63 × 10 6 , 1.54 × 10 6 ) exhibits a broader transparency window with the best fit provided by the ATS model. This agrees with the result in Fig. 5b,e . ( c ) At the transition region, both the EIT and the ATS models fit equally well to the transmission spectrum obtained for the mode pair with Q~(1.78 × 10 6 , 4.67 × 10 6 ). This agrees well with the results of Fig. 5c,f . Insets are enlarged versions of the spectra around the central frequency (zero detuning). Full size image As we showed in the previous sections and in the Supplementary Note 1 and Supplementary Fig. 1 , EIT/ATS model (intermediate-driving regime) has two terms, one of which is exactly the same as the ATS model (strong-driving regime) and the other is an interference term. We found theoretically and experimentally that and exhibit the same values because the contribution of the interference term is set to zero or to much lower values than the contribution from the ATS part during the curve-fitting because C 1 of equation (12) is a free-parameter ( Supplementary Note 2 and Supplementary Figs 4–6 ). Moreover, curve-fitting using the intermediate-driving regime model to the experimentally obtained transmission spectra revealed that for the transmission spectra for EIT case, the EIT/ATS model do not provide a good fit, although it has more free parameters. The discrepancy is significant around the zero-detuning where the transparency window exists. For the spectra obtained for the ATS and EIT-to-ATS transition, we see that the EIT/ATS model provides a curve-fitting at least as good as the ATS model ( Supplementary Note 2 and Supplementary Fig. 7 ). Although initially proposed, observed and used in atomic and molecular systems, Fano interference, EIT and ATS are among many quantum phenomena that have classical and, more importantly, all-optical analogues. Their demonstrations in on-chip physical systems using optical microresonators, metamaterials or plasmonics offer great promises for a wide range of applications including controlling the flow of light on-chip, high-performance sensors and studying the effects of many parameters that are difficult to test in atomic and molecular systems that need sophisticated and hard-to-access experimental environment and techniques. In particular, the capability of creating EIT and controlling the features of the transparency window in on-chip coupled optical microcavities is important for on-chip all-optical slowing and stopping of light, tunable optical filters, switching and nonlinear optics. Our approach, demonstrated in this work, provides a highly accessible and controllable platform that allows to test the effects of all relevant parameters (coupling strength, decay rates and frequency detunings) on the same coupled-resonator system for the observation and control of Fano resonances, EIT and ATS, as well as to probe the transitions among them. The capability to fine-tune the parameters at a high level, as demonstrated here, enabled us to show the avoided crossing in the ATS process as the frequency of one of the resonances were steered. In order to make good use of the observed transparency windows in coupled microresonators for the practical applications mentioned above, it is crucial that we know whether Fano interferences have played a role or not (that is, is the transparency the result of EIT or ATS?). Here we applied an objective test to characterize the parameters involved in Fano, EIT or ATS processes in coupled optical resonators and clearly discerned between EIT and ATS. The test used here is the AIC proposed by Anisimov et al. [17] This test clearly and with high confidence revealed whether the EIT or the ATS was involved in the experimentally obtained transmission spectra under different operating conditions. In addition to its capability to discriminate between EIT and ATS, the test revealed the sensitivity of the parameters involved. Our study demonstrates the suitability of the AIC method to characterize EIT and ATS in coupled microresonator systems and to study the effects of the system parameters on the observed spectra in the transition regime. How to cite this article : Peng, B. et al. What is and what is not electromagnetically induced transparency in whispering-gallery microcavities. Nat. Commun. 5:5082 doi: 10.1038/ncomms6082 (2014).